Human gut microbiota community structures in urban and rural populations in Russia The microbial community of the human gut has a crucial role in sustaining host homeostasis. High-throughput DNA sequencing has delineated the structural and functional configurations of gut metagenomes in world populations. The microbiota of the Russian population is of particular interest to researchers, because Russia encompasses a uniquely wide range of environmental conditions and ethnogeographical cohorts. Here we conduct a shotgun metagenomic analysis of gut microbiota samples from 96 healthy Russian adult subjects, which reveals novel microbial community structures. The communities from several rural regions display similarities within each region and are dominated by the bacterial taxa associated with the healthy gut. Functional analysis shows that the metabolic pathways exhibiting differential abundance in the novel types are primarily associated with the trade-off between the Bacteroidetes and Firmicutes phyla. The specific signatures of the Russian gut microbiota are likely linked to the host diet, cultural habits and socioeconomic status. The human gut microbiota represents the ‘last discovered organ’ of the human body [1] , showing functions ranging from digestion and protection against pathogen colonization to host immunity and central nervous system regulation. Its composition is influenced by genetics, the mode of delivery, diet, lifestyle, medical treatments and other factors [2] . The elucidation of global microbiota diversity is important for understanding the role of the microbiota in host health and for discovering ways to modulate the microbial community for disease prevention and treatment. Culture-independent methods, such as high-throughput DNA sequencing, provide insight into the total genomic composition (metagenome) of samples from both taxonomic and metabolic perspectives. Recently, several studies have produced large metagenomic data sets for the gut microbiota of populations from different countries. A catalogue of prevalent gut microbial genes was derived from the metagenomic analysis of stool samples obtained from 124 European individuals [3] . Long-term diet was found to be one of the significant factors linked to microbiota composition in US subjects [4] . Functions and structure of human gut microbiota were determined in a large cohort of US population [5] . Distinctions in microbiota composition were discovered between European, United States, African and Amerindian populations [6] , [7] . Other national metagenomic initiatives include Irish [8] , Korean [9] and Chinese [10] populations. However, metagenomic studies performed in Russia are underrepresented. In this study, we conduct a descriptive analysis of the gut microbiota of several diverse parts of Russian population using whole-genome sequencing. Although taxonomic analysis shows that the prevalent bacterial taxa are similar to those found in Western European and North American populations, we discovered novel community structures (dominated by Firmicutes and Actinobacteria) in healthy gut samples from Eastern Russia and rural regions. Gene repertoire analysis demonstrates that the novel community structures observed in the Russian metagenomes are distinctly enriched in functional pathways associated with Gram-positive Firmicutes. We suggest that further exploration of metagenomes in rural and remote areas will reveal even broader variation in community structures, representing historically stable variants of microbiota diversity before the widespread consumption of industrial food and antibiotics. Examination of the Russian microbiota We characterized the microbial communities of adult individuals living in metropolitan ( n =50) and rural ( n =46) areas by analysing stool samples (for the subject enrolment criteria, see Methods). The sampling geography covered a substantial part of the densely populated territory of Russia, including areas in Europe and south of Siberia ( Fig. 1a ). The urban settlements were represented by four of the top ten most populated cities in Russia (Saint Petersburg, Saratov, Rostov-on-Don and Novosibirsk), whereas the rural centres were represented by eleven villages and small towns in the Tatarstan, Omsk, Tyva and Khakassia regions. The average subject age was 36±18 years (mean±s.d. ), and the sexes were equally represented (48 females, 48 males) (for detailed metadata, see Supplementary Data 1 ). 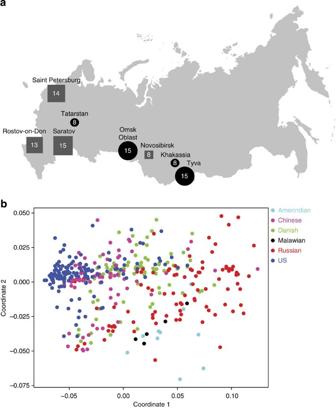Figure 1: Country-wide sampling highlights distinct features of Russian gut microbiota. (a) Sampling sites in Russia (n=8). Square and round bullets denote urban and rural areas, with the corresponding size and number inside representing the number of samples obtained at the site. (b) Two dimensional non-metric multidimensional scaling plot based on modified weighted UniFrac metric reveals a gradient structure of taxonomic composition in which Chinese (magenta) and Danish (green) occupy intermediate positions between Russian (red) and US (blue) samples. Two outliers (SAR_274 and NOV_283) with high proportions ofMethanobrevibacter,AkkermansiaorEscherichia/Shigellawere excluded. Figure 1: Country-wide sampling highlights distinct features of Russian gut microbiota. ( a ) Sampling sites in Russia ( n =8). Square and round bullets denote urban and rural areas, with the corresponding size and number inside representing the number of samples obtained at the site. ( b ) Two dimensional non-metric multidimensional scaling plot based on modified weighted UniFrac metric reveals a gradient structure of taxonomic composition in which Chinese (magenta) and Danish (green) occupy intermediate positions between Russian (red) and US (blue) samples. Two outliers (SAR_274 and NOV_283) with high proportions of Methanobrevibacter , Akkermansia or Escherichia/Shigella were excluded. Full size image The metagenomic composition of the microbiota was investigated via high-throughput shotgun sequencing using a SOLiD 4 sequencer, which produced 2.7±1.1 Gbp of 50 bp reads. The taxonomic and functional compositions of the samples were determined by mapping the reads against reference sets of microbial genomes and genes, respectively (details, including methodological validation, are described in the Methods and Supplementary Note 1 ). De novo assembly did not reveal any novel high-abundance taxa in the Russian metagenomes (see Methods). To check for distinctive features of the Russian metagenome composition in a global context, we performed a comparative analysis using existing sets of human gut shotgun reads from urban adult populations from Western Europe [3] (Denmark, n =85) and North America [4] (United States, n =137), rural communities from South America (Venezuela, n =10) and Africa [5] (Malawi, n =5), and 70 healthy subjects from China [9] . The applied DNA extraction and sample preparation methods were similar in all of these studies (see Methods). To evaluate the variation in the shotgun metagenomic composition across multiple sequencing platforms, we sequenced a subset of the Russian metagenomes using the SOLiD, Ion Torrent, 454 and Illumina platforms. The subsequent composition analysis produced highly correlated taxonomic profiles (see Supplementary Note 2 ), thus supporting the validity of comparisons between studies. Although the fraction of identified reads was similar between the Russian and non-Russian groups ( Supplementary Data 2 and Supplementary Note 3 ), the abundances of a number of microbial taxa were significantly different ( Supplementary Figs S1 and S2 , and Supplementary Data 3 ). Significant differences were found between the gut microbial communities of the Russian and the US, Danish and Chinese groups ( Fig. 1b ) via analysis of similarities (ANOSIM) [11] using a modified weighted UniFrac [12] metric (pair-wise ANOSIM, R =0.74, 0.50 and 0.26, respectively; P =9.999 × 10 −5 , 10,000 permutations, see Supplementary Table S1 ). A hierarchical representation of global diversity is shown in Supplementary Fig. S3 . Original microbial community structures in Russian samples The diversity of Russian metagenomes ( Supplementary Fig. S4 ) includes microbial communities that lack Prevotella or Bacteroides dominance; these two genera are ‘drivers’ of two of the three enterotypes [13] . Almost two-thirds of the Russian samples were not dominated by either of these genera (which is a higher fraction by 3.8±7.1 (median±s.d.) times than in the other populations (see Supplementary Table S2 ). Some of these mixed-type Russian metagenomes contained novel community structures that were not observed in non-Russian metagenomes. To assess the dominant taxa in these communities, sets of three of the most abundant genera were selected from each sample. For 92% of the combined metagenomes, more than 50% of the total abundance was contributed by these triplet sets. Approximately half (43 of 96) of the Russian metagenomes were dominated by triplets that were not found in non-Russian groups (see Supplementary Data 4 ). The majority of the triplets belonged to Firmicutes, followed by Bacteroidetes, Verrucomicrobia, Actinobacteria, Proteobacteria and Tenericutes, as well as Archaea. At a more detailed level, the novelty of the Russian metagenome composition was supported by the mean UniFrac distance from the non-Russian samples, which was significantly greater than that from the other Russian samples (Mann–Whitney’s one-sided test, P =1.202 × 10 −9 ). Sequencing of a variety of Russian metagenomes ( n =5) on both the SOLiD and Illumina platforms confirmed that the sets of three dominant genera were stable across different sequencing technologies (93% of the genera in triplets were preserved). For several samples, we discovered that the most abundant genus was unusual, that is, Bifidobacterium , Megamonas , Phascolarctobacterium , Lactobacillus or Akkermansia. Among other communities with unusual ‘drivers’, a number of the samples contained a high fraction of Escherichia coli . Differences in the corresponding genome-wise compositions suggested that this finding was not associated with laboratory contamination. One sample (Spb_73_13P) was dominated by a bacterium related to pathogenic Streptococcus infantarius subsp. infantarius BAA-102 (18.7% of the total abundance). Archaea were also distinctive contributors: although the major member of this group, Methanobrevibacter smithii , was generally more abundant in the Russian population than in all non-Russian cohorts, except the Amerindian group (Mann–Whitney’s one-sided test, P ≤0.00995), it was included in the top triplet in two of the Russian samples, showing abundances as high as 11.25% and 13.85%. Compact distinct subgroups share rural origins To explore the substructure of the microbiota diversity in the Russian samples, we searched for dense subgroups (showing similar structures). Significant cluster mining with bootstrapping using the R package pvclust [14] identified several subgroups with typical bacterial community structures ( Supplementary Figs S5, S6 ). Interestingly, each of the three largest subgroups mostly corresponded to a single rural area, that is, the Omsk, Tatarstan or Tyva regions ( Fig. 2 ). For each subgroup, 67–100% of the samples were dominated by the novel most-prevalent genus triplets. 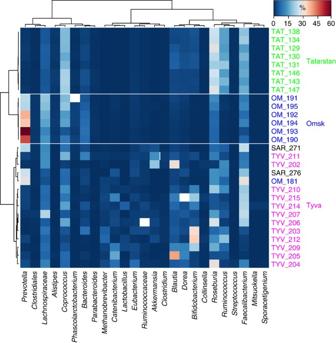Figure 2: Hosts from the same villages form subgroups with similar microbiota. Heat map showing the relative abundance of major genera (contributing >1% of the total abundance in at least one sample) for three compact subgroups, which are separated by white lines. Clustering was performed using a Spearman’s correlation-based dissimilarity metric and Ward linkage. Row-side label colours denote the samples from the prevalent regions: green–Tatarstan, blue–Omsk, magenta–Tyva and black–other. Figure 2: Hosts from the same villages form subgroups with similar microbiota. Heat map showing the relative abundance of major genera (contributing >1% of the total abundance in at least one sample) for three compact subgroups, which are separated by white lines. Clustering was performed using a Spearman’s correlation-based dissimilarity metric and Ward linkage. Row-side label colours denote the samples from the prevalent regions: green–Tatarstan, blue–Omsk, magenta–Tyva and black–other. Full size image A specific feature found in the Omsk subgroup was that it consisted of six of seven related metagenomes from the same family living in one village. The major genera identified in this group were Prevotella (36.6±13.4%; mean±s.d. ), Lachnospiraceae (15.3±3.2%), Coprococcus (13.1±5.5%) and Faecalibacterium (7.9±2.7%), indicating a community structure resembling the Malawian and Amerindian metagenomes. The similarity between the cluster samples varied with the choice of distance metric applied: the bacterial proportions were similar based on Spearman’s correlation (0.97±0.02, mean± s.d., with a pair-wise correlation across Russian samples of 0.78±0.07), but the UniFrac distance between the samples was quite high (0.03±0.02, with a mean of 0.07±0.03 across all Russian samples). This dependence of the similarity on the distance metric employed demonstrates that family metagenomes share genus compositions with similar ranks of abundance, as influenced by common genetics and past environmental exposure, consistent with a previous study of family metagenomes [5] . However, the quantitative proportions of genera may vary significantly depending on other variables. In the Tatarstan subgroup, all eight samples belonged to rural residents of this region. The community structure was characterized by the prevalence of Roseburia , Coprococcus , Faecalibacterium and Ruminococcus genera of the Firmicutes phylum (each forming 15–25% of the relative abundance), which were primarily contributed by the reference genomes Eubacterium rectale , Coprococcus eutactus , Faecalibacterium prausnitzii and Ruminococcus bromii , respectively. No similarity in community structures with non-Russian samples was observed during our meta-analysis (see Supplementary Table S4 ), suggesting that this represents an original subtype of microbiota within the Russian population. The third dense subgroup was dominated by samples from Tyva (12 of its 15 samples). Only three of the Tyva samples did not belong to the subgroup. The structure of these communities was defined by high proportions of Bifidobacterium (9.4±11.3%, mean±s.d., maximum 32.9%), which is more typical of infant microbiota [5] . At the genome level, the most abundant genus was represented by Bifidobacterium adolescentis , certain strains of which are reported to exhibit probiotic activity [15] . Moreover, this taxon was the most abundant genus in three of the samples, corresponding to a microbiota community type that was not observed in the non-Russian samples (except for a single Chinese sample dominated by Bifidobacterium breve ). The other bacterial genera in the Tyva subgroup were similar to those in the Tatarstan group. Microbiota in urban and rural populations The small number of samples for each geographic site and the specific age ranges and other metadata associated with each site confounded comparisons between separate geographic sites in Russia. However, when the samples were pooled by settlement size, the age and body mass index (BMI) distributions were generally not significantly different (Mann–Whitney’s two-sided test, P =0.5423 and 0.1316, respectively; see Fig. 3 ). There was no clear separation between the urban and rural metagenomes detected based on their taxonomic compositions (ANOSIM of UniFrac dissimilarity values, R =0.096, P =5 × 10 −4 , 10,000 permutations). The metagenomes from Russian cities were more similar to those of Western countries: despite equal representation of rural and urban populations, the original microbial community structures occurred in hosts from urban populations 2.6-fold less frequently than in the rural hosts (being found in 31 and 12 samples from these groups, respectively). The aforementioned compact subgroups were also found more often among rural populations, with only 2 of the 29 samples from these subgroups belonging to urban hosts. 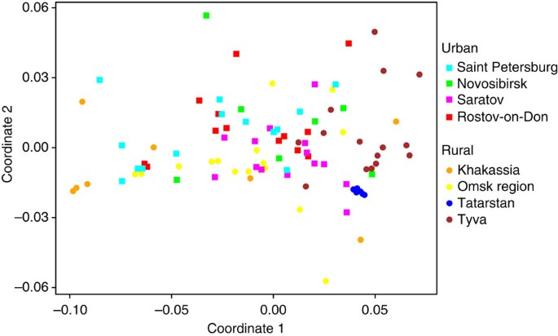Figure 3: Two dimensional non-metric multidimensional scaling (NMDS) plot of Russian metagenomes by taxonomic composition. UniFrac distances of 96 Russian samples were used in generating the NMDS. Point colour denotes sampling site, whereas shape denotes settlement size. Figure 3: Two dimensional non-metric multidimensional scaling (NMDS) plot of Russian metagenomes by taxonomic composition. UniFrac distances of 96 Russian samples were used in generating the NMDS. Point colour denotes sampling site, whereas shape denotes settlement size. Full size image Taxonomic typing of the Russian microbiota Cluster analyses of human gut microbial metagenomes are somewhat controversial. Although some studies demonstrate the existence of discrete categories of bacterial communities (enterotypes) [6] , [9] , [13] , [16] , others suggest that the distribution of bacterial components is more likely to exhibit a smooth, continuous structure [5] , [17] . In view of this ongoing discussion, we applied a cluster analysis based on enterotypes methodology to determine whether the observed Russian metagenomic diversity could be divided into distinctive clusters. Several common dissimilarity measures were used to generate the clusters ( Supplementary Data 5 ). For each metric, the optimal number of clusters was determined using the Calinski–Harabasz index and was assessed with multiple cluster quality metrics, including the average silhouette width (ASW), predictive strength [18] and comparison with randomized simulated communities [13] (see Methods). Overall, although the optimal number of clusters varied from two to three, all of the clusterings only achieved moderate support, as determined by the ASW value ( Supplementary Table S3 ). Even the highest ASW value (from the UniFrac metric) was low (0.389). However, using various metrics, the ASW was shown to be two to three times higher than the mean ASW for randomized simulated communities (1,000 simulations of 96 samples), and the predictive strength was quite high ( Fig. 4 ). Interestingly, two clusters were obtained: the first was driven by the genus Prevotella , and the second exhibited a high representation of Bifidobacterium and various genera of the phylum Firmicutes. Thus, the previously reported cluster with a high abundance of Bacteroides [6] , [13] was not observed, and the contribution of this genus was not significantly different between the two clusters ( P =0.8857, Mann–Whitney’s test). The urban and rural metagenomes were distributed equally between the clusters: 53% of the first and 52% of the second cluster were urban. When non-Russians were added to the Russian samples, the analysis produced two clusters: the first was driven by Prevotella , Bifidobacterium and various Firmicutes (it included most Russian samples) and the second by Bacteroides ( Supplementary Data 5 ). 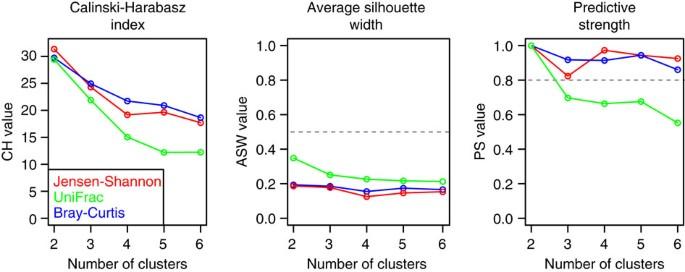Figure 4: Assessment of clustering quality for Russian cohort. There is a dependency between number of clusters in Russian cohort, calculated from three distance matrices (Bray–Curtis, UniFrac and Jensen–Shannon distances) and three quality indices: Calinski–Harabasz (CH), ASW and Prediction Strength (PS). The CH index is plotted, suggesting two as the optimal number of clusters for each distance matrix. For all of the metrics, the ASW values are rather low (below 0.5, which is the suggested threshold value for meaningful clustering5), although the prediction strength is high (above 0.8). The suggested thresholds are plotted in grey. Figure 4: Assessment of clustering quality for Russian cohort. There is a dependency between number of clusters in Russian cohort, calculated from three distance matrices (Bray–Curtis, UniFrac and Jensen–Shannon distances) and three quality indices: Calinski–Harabasz (CH), ASW and Prediction Strength (PS). The CH index is plotted, suggesting two as the optimal number of clusters for each distance matrix. For all of the metrics, the ASW values are rather low (below 0.5, which is the suggested threshold value for meaningful clustering [5] ), although the prediction strength is high (above 0.8). The suggested thresholds are plotted in grey. Full size image Rural subgroups and metabolic benefits to the host Analysis of the microbial drivers of the Tyva- and Tatarstan-dominated compact subgroups showed that they are prevalent in the healthy gut and complement mutual metabolism in ways that may be beneficial to host health. In particular, R. bromii , B. adolescentis and E. rectale are essential fermenters of type 2 and type 3 resistant starches [19] . During cocultivation in vitro , the first species significantly increases type 3 resistant starch utilization by the last two, having an essential role in the metabolism of these substrates, which have health benefits [20] . In addition, B. adolescentis is involved in metabolic cross-feeding with Roseburia and Eubacterium spp. bacteria through providing them with oligosaccharides released from complex substrates, as well as fermentation end products (lactate and acetate) [21] . High proportions of Coprococcus and Roseburia found in elderly people differentiate the microbiota of healthy community dwellers from long-term care patients, whereas the loss of Ruminococcus is associated with the transition to frailty [8] . Metabolomic analysis of fecal water have demonstrated that these species are associated with higher levels of butyrate [8] , which has an important role in gut homeostasis and integrity [22] . Another driver of the Tyva and Tatarstan metagenomes, F. prausnitzii , is a prominent butyrate producer [23] . F. prausnitzii , E. rectale and Roseburia spp. are prevalent in controls compared with type 2 diabetes patients [9] , and the latter two bacteria are more abundant in controls compared with atherosclerosis patients [16] . On the basis of the features of the novel communities found in the Tatarstan and Tyva populations, we suggest that these metagenomes provide examples of microbiota that promote human health. Comparative functional profiling In contrast to 16S rRNA sequencing, shotgun sequencing examines not only the taxonomic composition but also the total functional genetic potential of a microbial community. Thus, sequencing reads were aligned to the MetaHIT reference catalogue of prevalent human gut microbial genes, which contains 3.3 million sequences [3] , and were aggregated based on the Kyoto Encyclopedia of Genes and Genomes (KEGG) Orthology (KO) terms (see Methods). To determine significant large-scale variations in metabolism, we identified differentially abundant pathways using R package piano [24] for gene set enrichment analysis (see Methods). The Malawian and Amerindian groups were not considered in this part of the comparative analysis because of their low coverage depth and possible biases. The majority of the pathways that were differentially abundant in the Russian populations compared with the US and Danish groups coincided with the observed changes in the Bacteroidetes/Firmicutes ratio ( Supplementary Data 6 ). Enrichment of the following pathways was obviously linked to the higher levels of Firmicutes [25] , [26] : the phosphotransferase system and flagellar assembly (Russian versus Western) and ATP-binding cassette transporters (rural Russian versus urban Russian). The relative overrepresentation of the phosphotransferase system pathway in Russian metagenomes ( Fig. 5 ) corresponded to the fact that Firmicutes are more specialized towards oligosaccharides than Bacteroidetes, which possess a repertoire of degradation enzymes for a wide variety of carbohydrates [27] . In contrast, Bacteroidetes-abundant groups were enriched in glycosaminoglycan degradation, amino sugar and nucleotide sugar metabolism (United States, Danish and Chinese versus Russian) and lipopolysaccharide biosynthesis (urban Russian versus rural Russian and Chinese versus Russian). These effects reflect the wealth of genes encoding glycosaminoglycan degradation enzymes in the genomes of Gram-negative Bacteroides [27] , [28] . 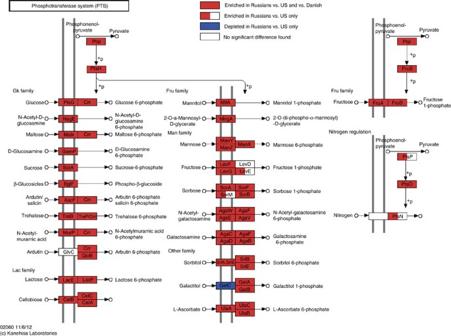Figure 5: Overrepresentation of phosphotransferase system genes in Russian samples compared with US and Danish samples. Overrepresented pathways were identified using Mann–Whitney’s one-sided test with false-discovery rate-adjustedP-values as described in Methods. The KO terms that are differentially abundant between the groups are indicated in colour. Figure 5: Overrepresentation of phosphotransferase system genes in Russian samples compared with US and Danish samples. Overrepresented pathways were identified using Mann–Whitney’s one-sided test with false-discovery rate-adjusted P -values as described in Methods. The KO terms that are differentially abundant between the groups are indicated in colour. Full size image The small number of differentially abundant pathways identified between taxonomically distinct groups suggests that although the dominant bacteria in the Russian metagenomes varied markedly, the total microbiome remained in functional equilibrium. This conclusion is supported by the enzyme-level functional similarity of the Russian samples (pair-wise Spearman’s correlation of KO abundance 0.92±0.03, mean±s.d.) underlying the observed taxonomic diversity (pair-wise correlation for genera abundance was 0.77±0.08). This finding of metabolic homeostasis is in agreement with previous studies [3] , [4] . Few cross-national comparative studies of gut microbiomes have been performed to date [5] , [10] , [17] , [29] . Shotgun sequencing-based comparisons of functional metabolic potential and genomic diversity are only beginning to appear [30] , [31] . In this study, we performed a descriptive analysis of gut microbiomes in the Russian population, and we demonstrated their unique properties in the global context of large metagenomic studies from both taxonomic and functional perspectives. The novel features of the Russian microbiomes included original gut microbial communities (driven by genera from the Firmicutes and Actinobacteria phyla, which are associated with a healthy intestine) and underrepresented Bacteroides -driven communities. We assessed potential factors that would confound the outcomes of comparative analyses based on the available metadata, including the sample preparation method, choice of sequencing platform, and subject age and BMI. Our analyses, performed using multiple sequencing technologies, suggested that the technical bias was minimal and that DNA extraction methods were similar in all studies (see Supplementary Note 2 , Methods). In particular, the original sets of three dominant genera discovered through SOLiD sequencing were almost completely reproduced using the Illumina platform, which is the most prevalent platform for whole-genome sequencing of human microbiomes. Analysis of the subjects’ age and BMI in the Russian versus non-Russian groups showed that the differences were small ( Supplementary Table S3 ) and could, therefore, not have confounded obvious phylum-level effects. We suggest that the observed differences in microbiota composition are due to differences in diet, lifestyle and environment. The ‘drivers’ of the novel Russian communities are predominantly bacteria from the Firmicutes and Actinobacteria phyla that are nutritionally specialized towards starch [27] . Some of the representative species in these groups ( R. bromii and E. rectale ) demonstrated an increase in fraction when resistant starch was introduced into the diet [32] . Presumably, the novel communities are supported by high consumption of starch-rich bread and potatoes, which are typical staple foods in rural Russia, and natural products that are available even to low-income socioeconomic groups from their household plots [33] , [34] . The underrepresentation of this special microbiota in Western cohorts is correlated with the reduced consumption of resistant starch in the West compared with developing countries and increased food industrialization [35] , [36] . The similarities between the microbiota of Russian city populations and those found in Western cities are presumably associated with higher social standards and a Western lifestyle, which is particularly reflected in the diet in the form of increased consumption of meat products and processed food. We speculate that the ‘drift from the land’, which is significant in modern Russia, contributes to the greater variety of microbiota found in each city (as the three most significant compact subgroups detected by pvclust contained few urban samples). Russia comprises more than 150 ethnic groups with diverse cultural and social traditions, and a significant part of the population lives in rural areas. Thus, even a limited assessment of microbiota composition, as performed in the present study, can reveal novel communities that have not been previously observed in large metagenomic studies in other countries. We expect that broader global sampling of the microbiota of local rural cohorts, including isolated communities, will identify even greater variability in gut microbial communities. As some of the identified novel communities are primarily composed of species associated with a healthy gut, this research is of significant interest for identifying indigenous configurations of human microbiota before food industrialization and modulating the functions of the microbiota in health and disease. Although our analysis of collective metabolic capabilities revealed few differences in metabolism between different data sets, suggesting that the human microbiota is functionally stable, we expect that the real degree to which the metabolic potential is utilized will be demonstrated via metatranscriptomic and metaproteomic studies, especially on the mucosa-associated colonies at the interface of host–microbe interactions. In conclusion, we conducted a whole-genome analysis of the gut microbiomes of healthy Russian population and demonstrated that the metagenomic data was comparable across the most prevalent sequencing platforms. These data were also compared with published large-scale studies. Although the set of dominant gut bacteria was similar to those found in other populations, we identified some unique community structures. This information deepens our understanding of healthy human microbiome ecology and serves as a reference point for future epidemiological studies and translational applications. Moreover, we examined the Russian microbiota from a functional perspective, and although our results agree with earlier studies showing functional homeostasis independent of taxonomic composition, we also observed certain signatures related to carbohydrate metabolism. We further suggested possible explanations linking diet and lifestyle with microbial community functions and, finally, we showed that studying gut bacterial communities across regional cohorts with distinctive sociocultural features extends our knowledge of the landscape of healthy human gut microbiome diversity. Subject enrolment criteria The Ethics Committee of the Research Institute of Physico-Chemical Medicine approved the study protocol. All participants provided written informed consent. Inclusion criteria: Male or female inhabitants of large Russian Federation cities with a prevalence of processed food in the diet, without intestinal dyspepsia symptoms, and who did not receive anti-inflammatory or antimicrobial therapy for at least 3 months before inclusion were included in the study. Male or female inhabitants of villages or small towns in the Russian Federation with a prevalence of natural food in the diet, without intestinal dyspepsia symptoms, and who did not receive anti-inflammatory or antimicrobial therapy for at least 3 months before inclusion were included in the study. Exclusion criteria: The exclusion criteria were as follows: age <18 years; no written informed consent; inability to follow verbal and written instructions; positive pregnancy test or breast feeding; serious concomitant diseases (cardiovascular, pulmonary, renal or hepatic failure, cerebral ischaemia, blood disorders, decompensated diabetes mellitus and so on); patients with oncologic diseases; patients who had undergone surgical procedures less than 3 months before inclusion; and alcohol, toxin or drug abuse. Dietary notes No update of diet or cancellation of medical preparations was prescribed, with the exception of seven subjects (read sets Spb_66_6P, Spb_72_12P, Spb_74_14P, Spb_76_16P, Spb_100_40P, Spb_103_43P and Spb_105_45P), who were advised to eat more vegetables/fruit for half a year and who took extruded bran fermented with Saccharomyces cerevisiae (18 g daily) for 2–3 weeks before stool collection. Stool sample collection The patients did not take sorbents or laxatives (including magnesia and castor oil) before sample collection. Stool samples were collected in the absence of urine and toilet paper. Using a special spoon, a stool sample of ~10–20 g was placed in a sterile plastic container and immediately frozen at −20 °C. The frozen samples were stored at −20 °C and transported to the laboratory on dry ice. DNA extraction Total DNA was extracted using a modified standard method [37] . Fecal samples were thawed on ice, and 150 mg of sample was transferred into a new 2.0-ml tube. Next, 300 mg 0.1 mm zirconia/silica beads, 100 mg 0.5 mm zirconia/silica beads (BioSpec Products, USA) and 1,200 μl warm (30 °C) lysis buffer (500 mM NaCl, 50 mM Tris HCl pH 8, 50 mM EDTA, 4% SDS) were added to the tube. The tube was vortexed and the contents were homogenized by shaking on a Mini BeadBeater 16 (BioSpec Products) for 3 min with maximum intensity. The homogenized sample was incubated at 70 °C for 15 min and vortexed periodically. The tube was centrifuged for 20 min at 22,000 r.c.f. The supernatant was recovered into a new 2.0-ml tube and stored at 4 °C. The pellet was washed with 1,200 μl of lysis buffer, and the homogenization and centrifugation steps were repeated. The supernatant was added to the first supernatant in the same 2.0-ml tube. Nucleic acids were precipitated by the addition of 2 vol of ethanol and 1/10 vol sodium acetate for 1 h at –20 °C, followed by centrifugation for 20 min at 22,000 r.c.f. The pellet was washed with 1,000 μl of 80% ethanol and centrifuged again. The pellet was resuspended and pooled in 400 μl of TE buffer. After additional centrifugation for 15 min at 22,000 r.c.f., the supernatant was recovered into a new 2.0-ml tube with 1 μl RNase A solution (5 mg ml −1 ) and incubated for 1 h at 37 °C. The quality of the extracted DNA was evaluated by running 5 μl of purified DNA on a 1.0% agarose gel. The DNA quantity was evaluated with a Qubit fluorimeter (Invitrogen, USA). DNA sequencing Fragment DNA library construction and shotgun sequencing for the SOLiD 4 platform (Life Technologies, Foster City, CA, USA) were performed, according to the manufacturer’s instructions using the following kits: SOLiD Fragment Library Construction Kit, SOLiD Fragment Library Barcoding Module 1–16, SOLiD EZ Bead TM E80 System Consumables and SOLiD ToP Sequencing Kit, MM50/5. The resulting read length was 50 bp. Fragment DNA library construction and shotgun sequencing for the Ion Torrent PGM platform (Life Technologies) were performed, according to the manufacturer’s instructions, using the following kits: Ion Xpress Plus Fragment Library Kit, Ion OneTouch 200 Template Kit, Ion Sequencing 200 Kit and Ion 318 Chip Kit. Fragment DNA library construction and shotgun sequencing for the GS FLX+ platform (Roche, Basel, Switzerland) were performed, according to the manufacturer’s instructions, using the following kits: GS Rapid Library Prep Kit, GS Titanium SV emPCR Kit (Lib-L) v2, GS Titanium LV emPCR Kit (Lib-L) v2 and GS FLX Titanium Sequencing Kit XL+. Paired-end DNA library construction and shotgun sequencing for the HiSeq 2000 platform (Illumina, San Diego, CA, USA) were performed, according to the manufacturer’s instructions, using the following kits: TruSeq DNA sample prep kit v.2, TruSeq PE Cluster Kit v3-cBot-HS and TruSeq SBS Kit v3-HS. The resulting read length was 101 bp. De-multiplexing was performed using the CASAVA v. 1.8.2 software. Read pre-processing and alignment Colour-space reads lacking positions or median raw quality values less than QV=15 were discarded. To minimize sequencing errors, the resulting high-quality reads were subjected to error correction using Applied Biosystems SOLiD Accuracy Enhancement Tool (Foster City, CA) with previously published parameters [38] . This process was followed by quality-based trimming; all positions starting from the 5′-end were discarded until a high-quality position (QV≥30) occurred. Finally, reads shorter than 30 bp were discarded. SOLiD reads were mapped to a reference genome set and gene catalogue using Bowtie [39] alignment software. Each read was mapped without allowing for insertions/deletions, allowing three mismatches per read. The first two nucleotides were trimmed, resulting in a maximal mapped read length of 48 bp. A read with multiple possible mapping locations was mapped to one of the locations at random with an equal probability. Ion Torrent reads were aligned using Bowtie2 (ref. 40 ) software with the following parameters: -t -f -D 20 -R 3 -N 0 -L 20 -i S,1,0.50 --local. Before alignment to reference sets, the reads were filtered for human DNA, and reads that mapped to the human genome (version hg18) were discarded from further analysis. Taxonomic profiling Metagenomic reads were aligned to a reference catalogue consisting of genomes of bacterial and archaeal species known to inhabit the human gut. The reference genomes catalogue was composed of available genomes of known human gastrointestinal bacteria. The Human Microbiome Project catalogue was used as a primary source and was extended using genome lists from related studies [3] , [13] . Sequenced genomes of microbes found in the gastrointestinal tract were downloaded from the whole Human Microbiome Project project catalogue, and additional genomes were downloaded from the NCBI FTP site. A total of 444 genomes were obtained ( Supplementary Data 7 ). Genome coverage by read alignment was used to estimate the relative abundance of the corresponding genera in a metagenomic sample. As each read was mapped once at most and some genomes of closely related strains in the reference set display similar sequences, the genome coverage depth was summed across the corresponding genus, such that the resulting profile described the abundance of genera, rather than that of species or strains. The application of a previously proposed method based on unique clade-specific marker genes [41] resulted in highly correlated bacterial proportions (see Supplementary Note 1 ). Inference of relative genus abundance from coverage For each alignment of a read set to a reference genome or gene, two measures of coverage were extracted from BAM files using BEDtools software: the summary length of reads mapped to the reference and the fraction of the reference length covered by at least one read (coverage breadth). The breadth of genomic coverage was used to determine the presence of an organism in the metagenome, and 1% of the genome length was employed as the presence threshold. For reference genes, no cut-off was used, because the minimum length of trimmed reads (30 bp) exceeded 4% of an average gene length (700 bp). For each genome from the reference set, the coverage was normalized to the sequence length and the total read length of the sample (see equation (1)). The calculated genome coverage was aggregated across genera to obtain a genus coverage profile ( Supplementary Data 8 ). For assessing the fraction of each genus for comparison, the genus abundance vector was normalized to a 100% sum for each sample. Weighted UniFrac metric modification for genome abundance A UPGMA tree of the reference genomes was constructed via multiple alignment of their 16S sequences using the MUSCLE [42] algorithm ( Supplementary Fig. S7 ). For each metagenomic sample, the relative genome abundance was assigned as a weight to the tree leaves (rather than operational taxonomic unit counts). Genomes showing zero abundance across all samples were excluded from the tree. If the 16S sequence was not available for a genome, its abundance was added to the leaf of the closest strain. The resulting tree was employed to calculate the weighted UniFrac distance between the samples using QIIME [43] . ANOSIM was performed with R software vegan package [44] . Sample clustering Clustering of taxonomic profiles was performed using the k -medoids algorithm (PAM clustering) with R statistical software [45] using seven dissimilarity metrics: the Spearman’s correlation-based, Euclidean, Manhattan, Canberra, Bray–Curtis, Jensen–Shannon divergence and UniFrac distances. Maximization of the Calinski–Harabasz index was performed to select the optimal number of clusters. The quality of clustering was assessed based on the ASW and predictive strength, and through comparison with the clustering of randomized simulated communities. The cluster analysis was performed using the R packages fpc [46] , cluster [47] and ecodist [48] . Identification of differentially abundant pathways For functional gene classification, the original KEGG annotations from the MetaHIT gene catalogue were used. Reads were aligned to the gene catalogue, and the relative abundance of each KO term was calculated as the total read length of the included catalogued reference genes normalized to total read lengths mapped to the whole catalogue. To identify KEGG pathways showing significantly different enrichment between the groups, the relative abundances of the included KO terms were compared using a Mann–Whitney one-sided test for each KEGG pathway. The resulting P -values were false-discovery rate adjusted and analysed using the R package piano, taking into account the direction of change for each KO abundance. The selected parameters included ‘reporter feature algorithm’ as the statistical gene set analysis method and ‘gene sampling’ as the significance assessment method. The significance threshold for directional P -values was 1 × 10 −3 ; for each group comparison, we selected only the pathways where at least half of the KO terms in the pathway were differentially abundant. In all analyses in which groups of samples were compared by settlement size (rural versus urban), samples from small towns were regarded as rural. De novo assembly and novel gene detection For each sample, quality-filtered reads were subjected to the SOLiD Accuracy Enhancement Tool error correction algorithm. The corrected reads were assembled de novo using SOLiD de novo tools, v2.2, with parameters adjusted for metagenomic reads [38] . Read assembly resulted in 3.4 Gbp contigs (35.8±15.8 Mbp per sample, mean±s.d., n =95). The assembly of one sample failed because of insufficient memory. The open reading frames in the contigs were detected using MetaGeneMark [49] and were translated. Protein sequences longer than 100 aa were aligned to the translated gene catalogue using BLASTP. The number of novel sequences (that did not match the gene catalogue with an e -value >0.001 and length >100) was 33,688. These sequences were extended using contigs assembled from reads that failed to map to the gene catalogue (with redundant sequences being removed). The resulting set contained 41,474 genes, representing 1.26% novel additions to the gene catalogue. Accession codes: Gut metagenome sequences have been deposited in the Sequence Read Archive under accession code SRA059011 . The contigs are available for download from the Russian Metagenome Project website ( http://www.metagenome.ru/files/rus_met/ ). How to cite this article: Tyakht, A.V. et al. Human gut microbiota community structures in urban and rural populations in Russia. Nat. Commun. 4:2469 doi: 10.1038/ncomms3469 (2013).